RhoA and ROCK mediate histamine-induced vascular leakage and anaphylactic shock Histamine-induced vascular leakage is an integral component of many highly prevalent human diseases, including allergies, asthma and anaphylaxis. Yet, how histamine induces the disruption of the endothelial barrier is not well defined. By using genetically modified animal models, pharmacologic inhibitors and a synthetic biology approach, here we show that the small GTPase RhoA mediates histamine-induced vascular leakage. Histamine causes the rapid formation of focal adherens junctions, disrupting the endothelial barrier by acting on H1R Gα q -coupled receptors, which is blunted in endothelial Gα q/11 KO mice. Interfering with RhoA and ROCK function abolishes endothelial permeability, while phospholipase Cβ plays a limited role. Moreover, endothelial-specific RhoA gene deletion prevents vascular leakage and passive cutaneous anaphylaxis in vivo , and ROCK inhibitors protect from lethal systemic anaphylaxis. This study supports a key role for the RhoA signalling circuitry in vascular permeability, thereby identifying novel pharmacological targets for many human diseases characterized by aberrant vascular leakage. The critical importance of the endothelial barrier integrity for vascular homeostasis is long well established [1] , [2] . Indeed, the breakdown of the endothelial barrier function, which can result in an uncontrolled increase in vascular permeability and vessel leakiness, contributes to oedema formation and inflammation in many pathological conditions [1] , [2] , [3] . Both, transcellular and paracellular mechanisms, the latter also referred to as intercellular, can mediate increased endothelial permeability [1] , [2] , [3] . While the transcellular passage of plasma molecules and cells often involves a complex system of vesiculo-vacuolar organelle transport, intercellular passage involves the dynamic opening and closure of endothelial cell–cell contacts by disrupting the adherens junctions that preserve the vascular barrier [1] , [2] , [3] . In endothelial cells, these adherens junctions are established and maintained by the interactions between vascular endothelial cadherin (VE-cadherin) in adjacent cells [2] , [4] . The intracellular region of VE-cadherin is anchored to the actin-based cytoskeleton through its associated proteins, including α- and β-catenin, and plakoglobin [5] . Increase in vascular permeability occurs under many physiological conditions, including wound repair, inflammation and thrombotic reactions, while disturbed adherens junctions is a characteristic of pathological conditions involving vascular leakage and inflammation [2] , [6] . These include many human diseases, such as tumour-induced angiogenesis, ocular diseases and anaphylactic and septic shock, which has prompted the growing interest in understanding the molecular mechanisms underlying aberrant vascular leakiness in disease. For example, focal efforts have been made to understand how VEGF (vascular endothelial growth factor) [7] , which was also described as a vascular permeability factor [8] , causes endothelial barrier disruption and vascular leakiness during normal and pathological angiogenesis. VEGF promotes endothelial cell survival, proliferation and migration by acting on its cognate cell surface tyrosine kinase receptor, VEGFR2 (Flk1, KDR) [9] . However, under pathological conditions excess of VEGF can cause plasma leakage and tissue oedema [7] , [8] . The emerging picture is that VEGF acts by a biochemical route that involves the sequential activation of VEGFR2 and the tyrosine kinase Src, and the concomitant tyrosine phosphorylation of VE-cadherin and the stimulation of a signalling pathway resulting in the activation of the small GTPase Rac1 (refs 2 , 10 ). In turn, these, and likely additional mechanisms, converge to promote the endocytosis of VE-cadherin complexes, thereby causing the disruption of the endothelial cell–cell junctions [2] , [10] . How other potent permeability factors act is much less understood. Among them, histamine plays a critical role in increased vascular permeability caused by multiple chronic and/or life-threatening inflammatory conditions, ranging from allergies and asthma to anaphylactic shock [11] , [12] . Histamine has been historically used for the establishment of in vivo methods for the study of vascular leakage [13] ; however, its precise mechanism of action is still not fully defined. Histamine acts through its four cognate G protein-coupled receptors (GPCRs), H1R to H4R [11] , [14] . We first confirmed that histamine promotes endothelial permeability through H1R receptors. As most GPCRs coupled to heterotrimeric G proteins of the Gα 11/q family, H1R receptors stimulate the phospholipase C (PLC) β family, which hydrolyses phosphatidylinositol 4,5-bisphosphate to produce two second messengers: inositol 1,4,5-trisphosphate (IP 3 ) and diacylglycerol [15] . IP 3 raises cytoplasmic Ca 2+ levels, which stimulates multiple calcium-regulated mechanisms, and together with diacylglycerol, activates classic Protein Kinase C isozymes (PKCs) [16] . However, Gα q can also interact directly with a large number of downstream molecules, including serine-threonine and tyrosine kinases, guanine nucleotide-exchange factors (GEFs) for Rho GTPases, scaffolding molecules and tetratricopeptide repeat-containing proteins [15] , [17] , many of which could play a role in histamine-induced vascular permeability. Here, we show that endothelial-specific Gα 11/q gene deletion prevents histamine-induced vascular leakage. However, the activation of PLCβ and the consequent generation of diffusible second messengers play only a limited role in endothelial permeability. Instead, the activation of RhoA by histamine is essential for the disruption of the endothelial barrier function in vitro and for the promotion of vascular leakiness in vivo . At the molecular level, we show that histamine stimulates a Rho GEF, Trio, acting downstream from Gα q , which in turn promotes the activation of RhoA and its regulated signalling circuitry, including the serine-threonine kinase ROCK. This results in the formation of focal adherens junctions (FAJs) and the disruption of the endothelial barrier. Ultimately, we provide evidence that RhoA activation is required for vascular permeability caused by histamine and other permeability factors released upon mast cell degranulation, and that inhibition of RhoA or its downstream target, ROCK, may represent suitable targets for pharmacological intervention in multiple disease conditions that involve aberrant vascular leakage. Limited role of PLCβ in histamine-induced permeability The precise molecular mechanisms by which histamine and other inflammatory mediators regulate endothelial permeability in vivo are still not fully understood. Histamine induced a rapid increase in vascular leakage in an in vivo live animal imaging system, which was dose dependent, as assessed further by the tissue extravasation of Evans blue (Miles assay) ( Fig. 1a–c ). This was recapitulated in in vitro endothelial permeability assays ( Fig. 1d ). Among the four G-protein-linked histamine receptors, the central role of H1R for histamine-induced endothelial permeability was confirmed using subtype-specific histamine receptor inhibitors ( Fig. 1e ). H1R couples to the Gα q G protein family, which activates PLCβ and the consequent accumulation of diacylglycerol and IP 3 , and increased intracellular Ca 2+ levels [14] . We verified the rapid histamine-induced cytosolic Ca 2+ accumulation in immortalized endothelial cells ( Fig. 1f ). In general, Gα 11 and Gα q play a redundant role in vivo [18] . Accordingly, combined knockdown of Gα 11 and Gα q ( Fig. 1g,h ) but not single Gα q family protein blocked histamine-induced permeability in vitro . Furthermore, Gα 11 deficiency combined with inducible gnaq ( Gα q ) gene excision in the endothelial cells ( Fig. 1i,j ) using the tamoxifen-inducible endothelial-specific Cdh5-CreERT 2 system [19] abolished histamine-induced permeability in vivo ( Fig. 1k ), the latter aligned with prior reports using tie2-Cre ERT 2 to excise Gα q in Gα 11 knockout (KO) mice [20] . 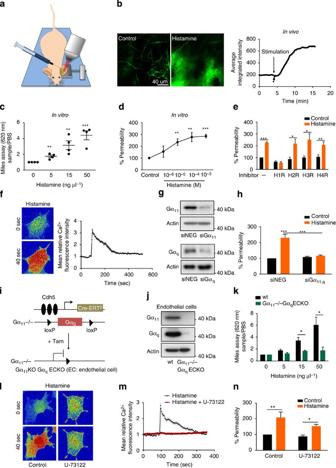Figure 1: Histamine-induced permeability is dependent on Gα11/q-coupled receptors but does not require PLC activation. (a) Schematic representation of live animal imaging of histamine-induced vascular leakage in the ear. (b) Mice were injected i.v. with 500 kDa FITC dextran and the ear skin was punched by a 29-gauge needle embedded in 10−4M histamine solution (see ‘Intravital imaging of vascular leakage in mouse ear skin’ in Methods) (repeated twice). (c)In vivopermeability assay: Evans blue extravasation was determined after subcutaneous injection of 20 μl of the indicated doses of histamine (n=4 per group). (d) Immortalized endothelial (EAhy926 cells) monolayers were challenged with histamine forin vitropermeability assay. Quantification of three independent experiments is shown (n=4 per group). (e) Cells were incubated with histamine receptor inhibitors (10 μM) 15 min prior to histamine (orange bars) addition. Quantification of two independent experiments is shown (n=4 per group). (f) Representative pictures and measurement of Ca2+fluorescence intensity after histamine (10−4M) stimulation. (g) Western blots (WBs) from endothelial cells treated with siRNA control (siNEG) or siRNA for Gα11and Gαq. (h) Combination of Gα11and GαqsiRNA was testedin vitroon histamine-induced permeability. Quantification of at least three independent experiments is shown (n=4 per group). (i) Schematic representation of theGα11knockout and endothelial-specific Gαq-deficient (ECKO) mice. (j) WBs from mouse lung endothelial cells from the indicated genetic backgrounds treated with 10 μM 4OH-Tamoxifen. (k) Evans blue extravasation was determined after subcutaneous injection of 20 μl of the indicated doses of histamine. Quantification of two independent experiments is shown (n=6 per group). (l,m) U-73122 (1 μM) treatment (where applied) 15 min prior to histamine stimulation. Representative pictures (l) and measurement (m) of Fluo-3 AM Ca2+indicator fluorescence intensity after histamine (10−4M) stimulation. (n) The effect of U-73122 (1 μM) was tested on histamine-induced permeability. Quantification of at least three independent experiments is shown (n=5 per group). Statistical significance was determined by an unpaired two-tailed Student’st-test. Data are represented as mean±s.e.m. *P<0.05; **P<0.01; ***P<0.001. Figure 1: Histamine-induced permeability is dependent on Gα 11/q -coupled receptors but does not require PLC activation. ( a ) Schematic representation of live animal imaging of histamine-induced vascular leakage in the ear. ( b ) Mice were injected i.v. with 500 kDa FITC dextran and the ear skin was punched by a 29-gauge needle embedded in 10 −4 M histamine solution (see ‘Intravital imaging of vascular leakage in mouse ear skin’ in Methods) (repeated twice). ( c ) In vivo permeability assay: Evans blue extravasation was determined after subcutaneous injection of 20 μl of the indicated doses of histamine ( n =4 per group). ( d ) Immortalized endothelial (EAhy926 cells) monolayers were challenged with histamine for in vitro permeability assay. Quantification of three independent experiments is shown ( n =4 per group). ( e ) Cells were incubated with histamine receptor inhibitors (10 μM) 15 min prior to histamine (orange bars) addition. Quantification of two independent experiments is shown ( n =4 per group). ( f ) Representative pictures and measurement of Ca 2+ fluorescence intensity after histamine (10 −4 M) stimulation. ( g ) Western blots (WBs) from endothelial cells treated with siRNA control (siNEG) or siRNA for Gα 11 and Gα q . ( h ) Combination of Gα 11 and Gα q siRNA was tested in vitro on histamine-induced permeability. Quantification of at least three independent experiments is shown ( n =4 per group). ( i ) Schematic representation of the Gα 11 knockout and endothelial-specific Gα q -deficient (ECKO) mice. ( j ) WBs from mouse lung endothelial cells from the indicated genetic backgrounds treated with 10 μM 4OH-Tamoxifen. ( k ) Evans blue extravasation was determined after subcutaneous injection of 20 μl of the indicated doses of histamine. Quantification of two independent experiments is shown ( n =6 per group). ( l , m ) U-73122 (1 μM) treatment (where applied) 15 min prior to histamine stimulation. Representative pictures ( l ) and measurement ( m ) of Fluo-3 AM Ca 2+ indicator fluorescence intensity after histamine (10 −4 M) stimulation. ( n ) The effect of U-73122 (1 μM) was tested on histamine-induced permeability. Quantification of at least three independent experiments is shown ( n =5 per group). Statistical significance was determined by an unpaired two-tailed Student’s t -test. Data are represented as mean±s.e.m. * P <0.05; ** P <0.01; *** P <0.001. Full size image The effect of histamine was recapitulated by a synthetic biology approach ( Supplementary Fig. 1a ). Immortalized endothelial cells were engineered to express a synthetic Gα q receptor (Sy-Rq, also known as DREADDs [21] , [22] ) ( Supplementary Fig. 1b ), which can be activated by clozapine N -oxide (CNO), an inert metabolite of clozapine. CNO treatment was sufficient to activate Ca 2+ release and endothelial permeability ( Supplementary Fig. 1c–e ) mimicking histamine. Accordingly, a small-molecule PLC inhibitor, U-73122, which elevated slightly the cytosolic Ca 2+ levels, blocked potently the histamine-induced Ca 2+ release ( Fig. 1l,m ). Surprisingly, however, PLCβ inhibition had a more limited impact on endothelial permeability ( Fig. 1n ). This was further confirmed with the synthetic biology approach ( Supplementary Fig. 1f–h ), suggesting that endothelial permeability caused by stimulation of Gα q -coupled receptors relies only partially on PLCβ activation. RhoA mediates histamine-induced endothelial permeability While Gα 11/q interaction and rapid activation of PLCβ has been extensively studied, Gα 11/q also stimulates multiple downstream molecules that can also interact with Gα 11/q (refs 15 , 17 ), and hence could contribute to the endothelial permeability. Among these Gα 11/q targets, we focused on the small GTPase RhoA, which is often associated with thrombin-induced permeability in vitro [23] . Endothelial thrombin receptors are coupled to Gα 12/13 proteins, but RhoA activation can also occur in response to Gα q -coupled receptors [24] . Indeed, histamine, and CNO in Sy-Rq-expressing endothelial cells, induced a rapid and persistent activation of RhoA ( Fig. 2a,b ; Supplementary Fig. 2a ). RhoA knockdown and RhoA inhibition by C3 toxin [25] had limited impact on basal endothelial leakage, but blocked histamine- and CNO-induced permeability ( Fig. 2c–e ). Aligned with our prior observations, combined Gα 11 and Gα q knockdown abrogated RhoA activation ( Supplementary Fig. 2b ), whereas the PLC inhibitor did not have an effect ( Supplementary Fig. 2c ). 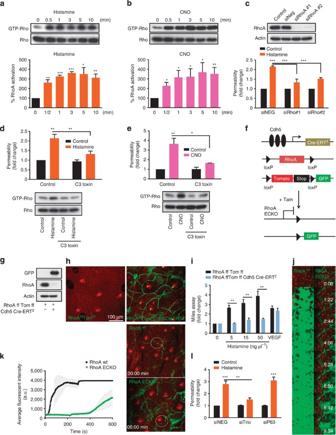Figure 2: RhoA activation is critical for histamine-induced permeability. (a,b) Time-course experiments of histamine (10−4M) (orange) or CNO (100 nM) (purple) stimulation in immortalized endothelial cells or endothelial Sy-Rq cells, respectively, and corresponding quantifications (n=3 per group). (c) Immortalized endothelial cells were treated with siRNA for RhoA and lysed for western blot (WB) or plated forin vitropermeability experiments. Quantification of at least three independent experiments is shown (n=5 per group). (d,e) Immortalized endothelial cells were incubated with C3 toxin (20 ng ml−1) for 16 h prior to histamine or CNO stimulation and were analysed for RhoA activation or used forin vitropermeability experiments. Quantification of three independent experiments is shown (n=3 per group). (f) Schematic representation of endothelial-specific RhoA-deficient (ECKO) mice with Tomato-GFP reporter. (g) Lung endothelial cells were isolated from RhoAf/fTomato-GFPf/fCdh5-CreERT2mice, treated with 4OH tamoxifen (10 μM) and lysed for WB analysis. (h) RhoAf/fTomato-GFPf/flittermates with/withoutCdh5-CreERT2were treated with tamoxifen, and fluorescence in the ears was evaluated by intravital microscopy. The intense red spots correspond to hair follicles that are surrounded by GFP+ blood vessels. (i) Evans blue extravasation was determined after subcutaneous injection of 20 μl of the indicated doses of histamine or 200 ng VEGF-A. Quantification of two independent experiments is shown (n=6 per group). (j) Mice were injected i.v. with 500 kDa FITC dextran and ear skin was punched using a 29-gauge needle embedded in 10−4M histamine solution. (k) Quantification of average fluorescent intensity. Under these low-magnification pictures the red colour represents the tdTomato fluorescence and the intense red spots correspond to hair follicles that are surrounded by GFP+ blood vessels in which FITC dextran circulates (n=5 regions per picture). The circles in the pictures are representative regions used for quantifications. (l) Immortalized endothelial cells were treated with control siRNA (siNEG) and siRNA for Trio (siTrio) or p63RhoGEF (siP63), as indicated and plated forin vitropermeability experiments. Quantification of at least three independent experiments is shown (n=5 per group). Statistical significance was determined by an unpaired Student’st-test. Data are represented as mean±s.e.m. *P<0.05; **P<0.01; ***P<0.001. Figure 2: RhoA activation is critical for histamine-induced permeability. ( a , b ) Time-course experiments of histamine (10 −4 M) (orange) or CNO (100 nM) (purple) stimulation in immortalized endothelial cells or endothelial Sy-Rq cells, respectively, and corresponding quantifications ( n =3 per group). ( c ) Immortalized endothelial cells were treated with siRNA for RhoA and lysed for western blot (WB) or plated for in vitro permeability experiments. Quantification of at least three independent experiments is shown ( n =5 per group). ( d , e ) Immortalized endothelial cells were incubated with C3 toxin (20 ng ml −1 ) for 16 h prior to histamine or CNO stimulation and were analysed for RhoA activation or used for in vitro permeability experiments. Quantification of three independent experiments is shown ( n =3 per group). ( f ) Schematic representation of endothelial-specific RhoA-deficient (ECKO) mice with Tomato-GFP reporter. ( g ) Lung endothelial cells were isolated from RhoA f/f Tomato-GFP f/f Cdh5-CreERT 2 mice, treated with 4OH tamoxifen (10 μM) and lysed for WB analysis. ( h ) RhoA f/f Tomato-GFP f/f littermates with/without Cdh5-CreERT 2 were treated with tamoxifen, and fluorescence in the ears was evaluated by intravital microscopy. The intense red spots correspond to hair follicles that are surrounded by GFP+ blood vessels. ( i ) Evans blue extravasation was determined after subcutaneous injection of 20 μl of the indicated doses of histamine or 200 ng VEGF-A. Quantification of two independent experiments is shown ( n =6 per group). ( j ) Mice were injected i.v. with 500 kDa FITC dextran and ear skin was punched using a 29-gauge needle embedded in 10 −4 M histamine solution. ( k ) Quantification of average fluorescent intensity. Under these low-magnification pictures the red colour represents the tdTomato fluorescence and the intense red spots correspond to hair follicles that are surrounded by GFP+ blood vessels in which FITC dextran circulates ( n =5 regions per picture). The circles in the pictures are representative regions used for quantifications. ( l ) Immortalized endothelial cells were treated with control siRNA (siNEG) and siRNA for Trio (siTrio) or p63RhoGEF (siP63), as indicated and plated for in vitro permeability experiments. Quantification of at least three independent experiments is shown ( n =5 per group). Statistical significance was determined by an unpaired Student’s t -test. Data are represented as mean±s.e.m. * P <0.05; ** P <0.01; *** P <0.001. Full size image The mechanisms controlling the endothelial barrier function in mature vessels may differ from those involved in promoting endothelial permeability in vitro [2] . Thus, to challenge the role of RhoA in vascular leakage in vivo , we used an inducible loss-of-function genetic approach to excise the RhoA gene in endothelial cells ( Fig. 2f ). Excision efficiency was monitored using the Tomato-green fluorescent protein (GFP) reporter mouse strain [26] ; GFP-expressing cells (green) can be visualized upon CRE-mediated gene recombination ( Fig. 2f ). In vitro , treatment of lung endothelial cells with 4OH-tamoxifen resulted in RhoA deficiency and GFP expression ( Fig. 2g ). The high excision efficiency in vivo was verified by live animal imaging of the dorsal skin of the ear ( Fig. 2h ). RhoA endothelial cell-specific deficiency in vivo did not affect VEGF-induced vascular permeability, but it was sufficient to abrogate histamine-induced vascular leakage, as judged by Miles assays ( Fig. 2i ) and by the limited and delayed extravasation of fluorescent dextran when monitored by intravital imaging ( Fig. 2j,k ). We next explored the nature of the GEFs mediating RhoA activation by histamine, focusing on Kalirin, Trio and p63RhoGEF, which can interact with Gα q proteins [27] . Kalirin is primarily expressed in the central nervous system [28] , while Trio and p63RhoGEF have wider expression patterns. p63RhoGEF protein was not detectable in endothelial cells ( Supplementary Fig. 2d ), and short interfering RNAs (siRNAs) did not affect histamine-induced permeability ( Fig. 2l ). Instead, Trio knockdown abolished RhoA activation in response to histamine and histamine-induced endothelial barrier disruption ( Fig. 2l ; Supplementary Fig. 2d ). Trio exhibits a C-terminal region by which it can bind to activated Gα q directly [22] . In line with this observation, activation of H1R1 by histamine led to the progressive plasma membrane accumulation of GFP-tagged Trio ( Supplementary Fig. 2e,f ). RNA sequencing analysis confirmed Trio’s dominant expression in primary endothelial cells ( Supplementary Fig. 2g ). LARG, a Gα 12/13 -stimulated GEF, can link H1R to RhoA in other cell types [29] . However, LARG deficiency [30] did not affect histamine-induced permeability in vivo ( Supplementary Fig. 2h ). Thus, Trio may represent the most likely RhoGEF linking histamine receptors to RhoA in endothelial cells. Trio exhibits an N-terminal and a C-terminal GEF, which activate Rac1 and RhoA, respectively [22] . Aligned with this, histamine induced a small increase in Rac1 but not Cdc42 in endothelial cells ( Supplementary Fig. 2i ). However, Rac1 knockdown ( Supplementary Fig. 2j ) did not affect histamine-induced permeability ( Supplementary Fig. 2k ), and treatment with ITX3, an inhibitor of the Trio N-terminal Rac-GEF [31] did not affect histamine-induced RhoA activation nor histamine-induced permeability ( Supplementary Fig. 2l,m ). Thus, whereas histamine and Trio can stimulate Rac1 downstream from Gα q in endothelial and other cellular systems [22] , [32] , the activation of RhoA appears to be more robust and sustained in endothelial cells, and the primary driver of endothelial cell permeability. Histamine induces FAJs through Rho–ROCK Angiogenic factors such as VEGF transiently remodel the adherens junctions through a coordinate process resulting in the endocytosis of VE-cadherin complexes [2] , [10] . This prompted us to examine the effects of histamine on VE-cadherin adhesive junctions. In primary endothelial cells, we did not observe VE-cadherin endocytosis, but instead histamine led to the rapid transition from stable junctions to active remodelling junctions connected to radial actin bundles perpendicular to VE-cadherin ( Fig. 3a,b ). These zipper-like structures are known as focal adherens junctions (FAJs), which are characterized by the presence of vinculin [33] . Vinculin clearly co-localized with the FAJs after histamine stimulation ( Fig. 3a ), linking the VE-cadherin adhesive complex to the tip of radial stress fibres formed in response to actomyosin contraction. In contrast, VEGF did not promote the rapid accumulation of radial actin bundles nor the formation of vinculin-containing FAJs. Instead, VEGF can stimulate FAJ formation only after prolonged stimulation, likely in an indirect fashion [33] , [34] . These findings are aligned with the possibility that histamine uses a distinct, RhoA-mediated mechanism to promote endothelial permeability. 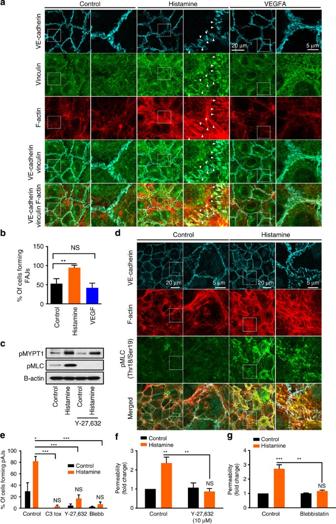Figure 3: Histamine induces focal adherens junction formation through the Rho-ROCK pathway. (a) HUVECs were treated with histamine (10 μM) (orange bar) or VEGF-A165(50 ng ml−1) (blue bar) for 10 min, immunostained with anti-VE-cadherin and anti-vinculin antibodies and stained with rhodamine-phalloidin to label F-actin. VE-cadherin, F-actin, vinculin and merged images are shown. The boxed areas are enlarged on the right side of the original images. White arrowheads point to FAJs. (b) The percentage of cells forming focal adherens junctions was quantified (n=30–40 cells per group). (c) HUVECs were treated with Y-27632 (10 μM) 30 min prior to histamine stimulation and 3 min after histamine treatment were lysed for western blot analysis. (d) HUVECs were treated with histamine, immunostained with VE-cadherin, pMLC antibodies and stained with rhodamine-phalloidin. VE-cadherin, F-actin, pMLC and merged images are shown. The boxed areas are enlarged on the right side of the original images. (e) The percentage of cells forming focal adherens junctions was quantified after treatment with C3 toxin (20 ng ml−1), Y-27632 (10 μM) and blebbistatin (10 μM) (n=30–40 cells per group). Immortalized endothelial cells were treated with Y-27632 (f) and blebbistatin (g) 30 min prior to histamine incubation and permeability was evaluated. Quantification of at least three independent experiments is shown (n=5 per group). Statistical significance was determined by an unpaired two-tailed Student’st-test. Data are represented as mean±s.e.m. NS, not significant; *P<0.05; **P<0.01; ***P<0.001. Figure 3: Histamine induces focal adherens junction formation through the Rho-ROCK pathway. ( a ) HUVECs were treated with histamine (10 μM) (orange bar) or VEGF-A 165 (50 ng ml −1 ) (blue bar) for 10 min, immunostained with anti-VE-cadherin and anti-vinculin antibodies and stained with rhodamine-phalloidin to label F-actin. VE-cadherin, F-actin, vinculin and merged images are shown. The boxed areas are enlarged on the right side of the original images. White arrowheads point to FAJs. ( b ) The percentage of cells forming focal adherens junctions was quantified ( n =30–40 cells per group). ( c ) HUVECs were treated with Y-27632 (10 μM) 30 min prior to histamine stimulation and 3 min after histamine treatment were lysed for western blot analysis. ( d ) HUVECs were treated with histamine, immunostained with VE-cadherin, pMLC antibodies and stained with rhodamine-phalloidin. VE-cadherin, F-actin, pMLC and merged images are shown. The boxed areas are enlarged on the right side of the original images. ( e ) The percentage of cells forming focal adherens junctions was quantified after treatment with C3 toxin (20 ng ml −1 ), Y-27632 (10 μM) and blebbistatin (10 μM) ( n =30–40 cells per group). Immortalized endothelial cells were treated with Y-27632 ( f ) and blebbistatin ( g ) 30 min prior to histamine incubation and permeability was evaluated. Quantification of at least three independent experiments is shown ( n =5 per group). Statistical significance was determined by an unpaired two-tailed Student’s t -test. Data are represented as mean±s.e.m. NS, not significant; * P <0.05; ** P <0.01; *** P <0.001. Full size image Histamine induced the rapid phosphorylation of the regulatory myosin light chain II (MLC), which was abolished by the ROCK inhibitor Y-27632 ( Fig. 3c ). Histamine also caused inhibitory phosphorylation on the myosin-binding subunit of MLC phosphatase 1 (MYPT1) ( Fig. 3c,d ), and ROCK inhibition led to a partial ( ∼ 35%) decrease of MYPT1 phosphorylation. Thus, while multiple kinases acting downstream of histamine receptors could be involved in the regulation of MYPT1 by phosphorylation [35] , ROCK is ultimately strictly required to initiate MLC phosphorylation. As a result, ROCK inhibition prevented the generation of contractile forces and stress fibres driving the formation of FAJs ( Fig. 3e ). Of interest, under basal conditions many endothelial cells exhibit few and often not fully developed FAJs, with few actin stress fibres attached to them, likely involved in dynamic junctional remodelling but with limited impact on intercellular permeability. Even these basal FAJs were nearly abolished by ROCK inhibition. Upstream inhibition of RhoA by C3 toxin and downstream inhibition of myosin II by blebbistatin had the same effect, preventing basal and stimulated FAJ formation ( Fig. 3e ). Consistently, ROCK inhibition abolished histamine- and CNO-induced endothelial permeability ( Fig. 3f,g ; Supplementary Fig. 3 ). ROCK inhibition protects from anaphylactic shock These observations provided an opportunity to translate these findings into potential clinical applications. Fasudil, a ROCK inhibitor currently being used in the clinic [36] , abrogated histamine-induced FAJs and endothelial permeability ( Fig. 4a–c ), as well as CNO-induced permeability ( Supplementary Fig. 4a ). Of direct translational relevance, mice pretreated with Fasudil were resistant to vascular leakage when challenged with histamine ( Fig. 4d ). 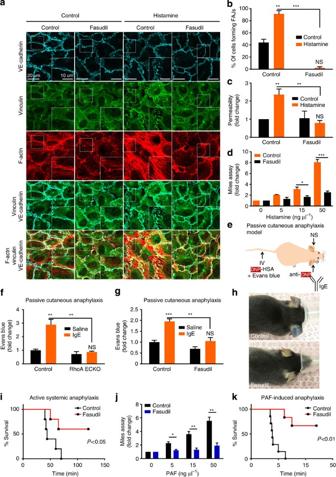Figure 4: Fasudil treatment prevents histamine- or PAF-stimulated vascular leakage and anaphylactic response. (a) HUVECs were treated with histamine for 10 min, immunostained with anti-VE-cadherin, anti-vinculin antibodies, and stained with rhodamine-phalloidin. VE-cadherin, F-actin, vinculin and merged images are shown, boxed areas are enlarged (right). (b) The percentage of cells forming focal adherens junctions was quantified after treatment with Fasudil (n=30–40 cells per group). (c) Endothelial monolayers were treated with Fasudil (10 μM) 30 min prior to histamine treatment (orange) and challenged for permeabilityin vitro.Quantification of at least three independent experiments shown (n=5 per group). (d) Mice were treated with normal saline or Fasudil (20 mg kg−1) by i.p. injection 2 h prior toin vivopermeability experiments. Evans blue extravasation was determined after subcutaneous injection of 20 μl of the indicated doses of histamine. Quantification of two independent experiments is shown (n=8 per group). (e) Schematic representation of the passive cutaneous anaphylaxis model. (f) Quantifications of Evans blue extravasation in ear biopsies correlate to the anaphylactic response in tamoxifen-treated RhoAf/fTom-GFPf/f(control) versus RhoAf/fTom-GFPf/fChd5Cre-ERT2(RhoA ECKO) littermates. Quantification of two independent experiments is shown (n=8 per group). (g,h) C57 mice were treated with PBS or Fasudil 2 h before the experiment. Evans blue extravasation was determined in ear biopsies and representative images are shown. Quantification of two independent experiments is shown (n=8 per group). (i) Survival of mice sensitized with BSA and challenged 14 days later with BSA was monitored for 2 h. Fasudil treatment took place 2 h before the challenge (n=5 per group). (j) Mice were treated with Fasudil (20 mg kg−1) by i.p. injection 2 h prior toin vivopermeability experiment. Evans blue extravasation was determined after subcutaneous injection of 20 μl of the indicated doses of PAF. Quantification of two independent experiments is shown (n=6 per group). (k) Survival of mice challenged with PAF i.v. injections was monitored for 2 h. Fasudil treatment took place 2 h before the challenge (n=7 per group). Statistical significance was determined by an unpaired Student’st-test or by the Mantel–Cox test for survival experiments. Data represented as mean±s.e.m. NS, not significant; *P<0.05; **P<0.01; ***P<0.001. Figure 4: Fasudil treatment prevents histamine- or PAF-stimulated vascular leakage and anaphylactic response. ( a ) HUVECs were treated with histamine for 10 min, immunostained with anti-VE-cadherin, anti-vinculin antibodies, and stained with rhodamine-phalloidin. VE-cadherin, F-actin, vinculin and merged images are shown, boxed areas are enlarged (right). ( b ) The percentage of cells forming focal adherens junctions was quantified after treatment with Fasudil ( n =30–40 cells per group). ( c ) Endothelial monolayers were treated with Fasudil (10 μM) 30 min prior to histamine treatment (orange) and challenged for permeability in vitro. Quantification of at least three independent experiments shown ( n =5 per group). ( d ) Mice were treated with normal saline or Fasudil (20 mg kg −1 ) by i.p. injection 2 h prior to in vivo permeability experiments. Evans blue extravasation was determined after subcutaneous injection of 20 μl of the indicated doses of histamine. Quantification of two independent experiments is shown ( n =8 per group). ( e ) Schematic representation of the passive cutaneous anaphylaxis model. ( f ) Quantifications of Evans blue extravasation in ear biopsies correlate to the anaphylactic response in tamoxifen-treated RhoA f/f Tom-GFP f/f (control) versus RhoA f/f Tom-GFP f/f Chd5Cre-ERT 2 (RhoA ECKO) littermates. Quantification of two independent experiments is shown ( n =8 per group). ( g , h ) C57 mice were treated with PBS or Fasudil 2 h before the experiment. Evans blue extravasation was determined in ear biopsies and representative images are shown. Quantification of two independent experiments is shown ( n =8 per group). ( i ) Survival of mice sensitized with BSA and challenged 14 days later with BSA was monitored for 2 h. Fasudil treatment took place 2 h before the challenge ( n =5 per group). ( j ) Mice were treated with Fasudil (20 mg kg −1 ) by i.p. injection 2 h prior to in vivo permeability experiment. Evans blue extravasation was determined after subcutaneous injection of 20 μl of the indicated doses of PAF. Quantification of two independent experiments is shown ( n =6 per group). ( k ) Survival of mice challenged with PAF i.v. injections was monitored for 2 h. Fasudil treatment took place 2 h before the challenge ( n =7 per group). Statistical significance was determined by an unpaired Student’s t -test or by the Mantel–Cox test for survival experiments. Data represented as mean±s.e.m. NS, not significant; * P <0.05; ** P <0.01; *** P <0.001. Full size image Histamine is not the only mediator released upon degranulation of mast cells after antigen recognition by immunoglobulin (Ig)E bound to mast cell FcɛRI receptors [12] . Therefore, we next used classical passive cutaneous anaphylaxis models to explore the role of endothelial RhoA in vascular leakage caused by mast cell degranulation ( Fig. 4e ) [20] . Endothelial-specific RhoA deficiency and Fasudil treatment were sufficient to prevent dye extravasation after local exposure to antigen in mice injected with anti-hapten-specific IgEs ( Fig. 4f–h ). Fasudil also protected from anaphylactic shock caused by active systemic anaphylaxis upon the injection of allergens [12] , [20] . All control-treated mice died within the first hour, whereas 60% of the Fasudil-treated mice survived ( Fig. 4i ). PAF promotes vascular permeability through Rho–ROCK The release of a platelet-activating factor (PAF) [37] by neutrophils stimulated by IgG antibody-antigen recognition is also involved in the anaphylactic response. PAF is a potent permeability factor that is also released in low amounts by mast cells concomitantly with histamine [12] . As PAF acts through Gα q -coupled receptors [20] , [38] , [39] , we investigated whether RhoA could also mediate PAF-induced vascular leakage. In vivo , PAF induced endothelial permeability in a dose-dependent manner ( Supplementary Fig. 4b ), likely by acting directly on PAF receptors on endothelial cells, and indirectly by promoting histamine release from mast cells [40] . In vitro , the direct PAF-induced endothelial permeability was mediated by RhoA ( Supplementary Fig. 4c ), while Fasudil treatment blocked PAF-induced permeability in vivo ( Fig. 4j ; Supplementary Fig. 4d ). Endothelial-specific RhoA deficiency was sufficient to protect from death from PAF-induced anaphylactic shock ( Supplementary Fig. 4e ). In turn, Fasudil-treated mice were protected from PAF-induced shock, as ∼ 72% of the mice survived, while all control-treated mice died within 1 h ( Fig. 4k ). Overall, our findings support a model whereby histamine and other permeability factors acting on Gα q -coupled GPCRs promote the activation of PLCβ and the rapid mobilization of calcium on endothelial cells, while a distinct Gα q downstream target, Trio, initiates the activation of RhoA and the consequent stimulation of ROCK ( Fig. 5 ). These two pathways converge to promote MLC phosphorylation and the stimulation of its contractile activity. Diffusible second messengers may promote MLC phosphorylation through Ca 2+ -induced myosin light chain kinase (MLCK) activation [35] , while in parallel, the protein–protein interaction-driven stimulation of RhoA by the association of Gα q with Trio may lead to MLC phosphorylation by ROCK. Concomitantly, ROCK and other yet to be identified kinases may inactivate MYPT1, thereby sensitizing MLC to the basal phosphorylating activity of MLCK even at normal intracellular calcium levels. The latter process, often referred to as ‘Ca 2+ sensitization’ [41] , [42] , may explain why the activation of RhoA appears to be dominant, as histamine-induced endothelial permeability relies partially on the PLCβ-initiated arm of the Gα 11/q signalling circuitry but it is strictly dependent on RhoA and ROCK function. Myosin II phosphorylation and activation may then cause the rapid redistribution of cortical actin into radial stress fibers anchored to VE-cadherin/catenin complexes through vinculin. Ultimately, the tension generated by actomyosin contraction promotes the relocalization of the VE-cadherin adhesion complexes to FAJs, and the formation of gaps disrupting the continuity of the endothelial barrier, thereby causing vascular leakiness ( Fig. 5 ). Whether the subsequent RhoA inactivation may be in turn required for barrier restoration under physiological conditions warrants further investigation. 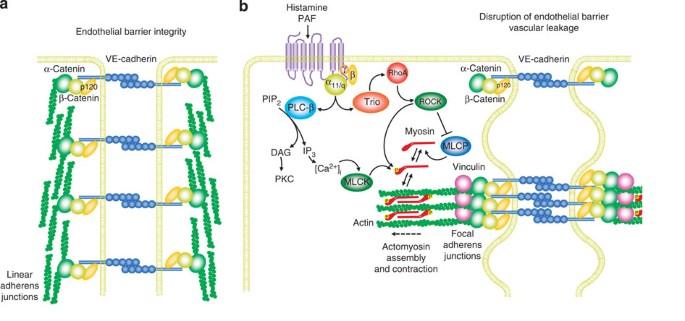Figure 5: Schematic representation of the mechanisms involved in endothelial cell permeability in response to histamine and PAF. Cartoon representing mature linear adherens junctions at steady state (a). The signalling circuitry disrupting the endothelial barrier function upon histamine or PAF activation (b). The tension generated by the RhoA-dependent actomyosin contraction promotes the relocalization of VE-cadherin adhesion complexes to focal adherens junctions and the consequent formation of gaps disrupting the continuity of the endothelial barrier, which results in increased endothelial permeability and vascular leakiness. See text for details. Figure 5: Schematic representation of the mechanisms involved in endothelial cell permeability in response to histamine and PAF. Cartoon representing mature linear adherens junctions at steady state ( a ). The signalling circuitry disrupting the endothelial barrier function upon histamine or PAF activation ( b ). The tension generated by the RhoA-dependent actomyosin contraction promotes the relocalization of VE-cadherin adhesion complexes to focal adherens junctions and the consequent formation of gaps disrupting the continuity of the endothelial barrier, which results in increased endothelial permeability and vascular leakiness. See text for details. Full size image An emerging picture from these studies is that RhoA activation plays a necessary and central role for endothelial permeability and vascular leakage when caused by histamine, PAF and mast cell degranulation. This information can now be exploited for therapeutic purposes with Fasudil and other ROCK inhibitors [43] . Fasudil has been shown to be effective for the treatment of systemic [44] and pulmonary hypertension [45] , [46] , stroke [47] , chronic heart failure [48] and to improve the prognosis of Alzheimer’s patients [49] . Its impact on atherosclerosis [50] , hypercholesterolaemia (NCT00120718) and Raynaud’s syndrome (NCT00498615) is under clinical evaluation. Thus, ROCK inhibition is emerging as a suitable pharmacological target in multiple human diseases. In this regard, although there is a risk that ROCK inhibition may exacerbate anaphylactic shock-induced hypotension, we found here that ROCK inhibitors may ultimately protect from death caused by systemic anaphylaxis and PAF. Overall, our present study suggests that Fasudil and other ROCK inhibitors may provide novel therapeutic approaches for a myriad of pathological conditions involving vascular leakage elicited by the acute release of vascular permeability factors, such in the allergic reaction and anaphylactic shock, whose risks and benefits would be worth pursuing in clinical trials. Cell lines and culture procedures The immortalized human endothelial cell line EAhy926 (ref. 51 ) (CRL-2922; ATCC) and HEK 293 (CRL-1573; ATCC) cells were maintained in DMEM supplemented with 10% fetal bovine serum (FBS) and 1 × antibiotic/antimycotic solution (Sigma-Aldrich). To establish immortalized endothelial cells (EAhy926) stably expressing Sy-Rq, cells were transfected with pCEFL-HA-Sy-Rq [22] using Lipofectamine-Plus (Invitrogen), according to manufacturer’s instructions, and selected by their ability to grow in 0.8 mg ml −1 G418 (A.G. Scientific). Positive haemagglutinin (HA)-expressing cells were sorted using a MoFlo legacy cell sorter (Beckman Coulter). Primary human umbilical vein endothelial cells were grown in endothelial cell medium EGM-2 BulletKit (Lonza). Isolation of mouse lung microvascular endothelial cells was performed as follows [52] : lungs were removed from two or more mice, washed in 10% FBS-DMEM, minced into 1–2-mm squares and digested with Collagenase Type I (2 mg ml −1 , Gibco) at 37 °C for 2 h with occasional agitation. The cellular digest was filtered through a 70-μm cell strainer, centrifuged at 1,500 r.p.m. and the cells were plated (day 0) on gelatin-coated dishes containing DMEM/F12 medium (Gibco) supplemented with 20% FBS, 100 μg ml −1 endothelial cell growth supplement (ECGS) (BD Biosciences) and antibiotics. On day 1, the floating cells including red blood cells were removed and washed with PBS and fresh culture medium was added. Dynabead sheep anti-rat IgG (Invitrogen) was incubated with a rat anti-mouse ICAM-2 mAb (3C4) (22.5 μl Ab per 150 μl dynabead solution) at 4 °C overnight and washed three times with PBS, 0.1% BSA and 2 mM EDTA. First purification using the pre-coated beads was done on day 5. After trypsinization, the bead-bound cells were recovered with a magnet, washed four times, resuspended in growth medium and then plated on fresh gelatin-coated dishes. On day 10, the cells were subjected to a second purification according to the same procedure. Purity (>85%) of endothelial cells was verified by PECAM-1 staining in FACS analysis. Endothelial cells were treated with 10 μM 4OH-tamoxifen for 10 days. Mice All animal studies were carried out according to NIH-approved protocols, in compliance with the Guide for the Care and Use of Laboratory Animals. All mice used were in C57BL/6 background, 8 weeks old or older and both males and females were used for experiments, except from LARG ko and littermates (mixed C57BL/6 and CD1 background). The generation of null alleles of the genes encoding Gα 11 (G nα11 ) and of the floxed alleles of the genes encoding Gα q ( Gnαq ) have been described previously [20] . The generation of the floxed alleles of the genes encoding RhoA has been described previously [53] . Endothelial-specific Gαq and RhoA knockouts were obtained by crossing the aforementioned mice with mice carrying a tamoxifen-inducible Cre-mediated recombination system driven by the Cdh5 promoter ( Cdh5-CreERT 2 ) [19] . Tamoxifen (3 mg per mouse per day in miglyol) was applied by intraperitoneal (i.p.) injections to 4–6–week-old mice for 5 consecutive days to induce Cre-mediated gene deletion. Larg knockout mice have been described previously [30] . Fasudil (20 mg kg −1 ) was applied by i.p. injections [54] 2 h before experiments. All experiments were conducted using littermate controls. siRNA, antibodies and reagents The following predesigned siRNAs were used: AllStars negative control, GNA11, Trio (Qiagen), GNAQ, p63RhoGEF (Santa Cruz Biotech Inc.) and RhoA (Invitrogen Inc.) ( Supplementary Table 2 ). The cells were transfected with control or targeting siRNA using Polyfect (Qiagen) or Lipofectamine RNAiMAX (Invitrogen) according to the manufacturer’s instructions. The following antibodies were used: rabbit anti-GNA11 (D-17; Santa Cruz Biotech), rabbit anti-GNAQ (C-19; Santa Cruz Biotech), mouse anti-HA (Covance), rabbit anti-RhoA (2117; Cell Signaling Technology), rabbit anti-GFP (D5.1; Cell Signaling Technology), rabbit β-actin (4967; Cell Signaling Technology), rabbit pMLC(Thr18/Ser19) (3674; Cell Signaling Technology), rabbit anti-VE-cadherin (D87F2; Cell Signaling Technology), mouse anti-vinculin (V9131; Sigma-Aldrich), rat anti-mouse ICAM-2 mAb (3C4; BD Pharmingen), rabbit anti-Trio (H120; Santa Cruz Biotech), goat anti-p63RhoGEF (G-14; Santa Cruz Biotech), Rhodamine-phalloidin (Invitrogen), Alexa Fluor 488- or Alexa Fluor 633-labelled goat anti-mouse and anti-rabbit IgG (Invitrogen), HRP-coupled goat anti-mouse and anti-rabbit IgG and rabbit anti-goat IgG (Southern Biotech). Santa Cruz Antibodies were used in 1:500 dilution and the rest were used in 1:1,000 dilution. Secondary antibodies for western blot were used in 1:50,000 and secondary antibodies for immunofluorescence were used in 1:500 dilution. Histamine, diphenhydramine, ranitidine, ciproxifan, JNJ7777120, PAF, Evans blue, anti-dinitrophenol-IgE (anti-DNP-IgE), DNP human serum albumin (DNP-HSA), BSA, CNO, U-73122, Y-27632, tamoxifen and 4OH-tamoxifen were obtained from Sigma-Aldrich. VEGF [7] was purchased from PeproTech Inc. Fluo-3/AM probe was purchased from Molecular Probes. Dynabead sheep anti-rat IgG was purchased from Invitrogen. Collagenase Type I was purchased from Gibco. Collagen Type I and ECGS were purchased from BD Biosciences. Miglyol 812N was purchased from Cremer Oleo GmbH&Co. Pertussis toxin and C3 toxin were purchased from List Biological Laboratories. Fasudil was purchased from LC Laboratories. Osmium tetroxide, 2.5% paraformaldehyde/glutaraldehyde in 0.1 M sodium cacodylate and hexamethyldisilazane buffers were purchased from Electron Microscopy Sciences. Ketamine and xylazine were purchased from NIH pharmacy. Immunoblot analysis The cells were lysed in lysis buffer (50 mM Tris-HCl, 150 mM NaCl, 1% Nonidet P-40) supplemented with protease inhibitors (0.5 mM phenylmethylsulfonyl fluoride, 10 μg ml −1 aprotinin and 10 μg ml −1 leupeptin). Equal amounts of proteins were subjected to SDS–polyacrylamide gel electrophoresis and transferred onto an Immobilon P, polyvinylidene difluoride membrane (Millipore, Billerica). The membranes were then incubated with the appropriate antibodies, mentioned above. The antigens were visualized using the Immobilon Western Chemiluminescent HRP substrate (Millipore) according to the manufacturer’s instructions ( Supplementary Fig. 5 ). The protein levels that corresponded to the immunoreactive bands were quantified using the ImagePC image analysis software (Scion Corp., Frederick, MD). Rho GTPase pulldown assay Rho activation in cultured cells was assessed as follows [30] : after serum starvation for 3 h, the cells were treated as indicated and lysed on ice in a buffer containing 20 mM Hepes, pH 7.4, 0.1 M NaCl, 1% Triton X-100, 10 mM EGTA, 40 mM β-glycerophosphate, 20 mM MgCl 2 , 1 mM Na 3 VO 4 , 1 mM dithiothreitol, 10 μg ml −1 aprotinin, 10 μg ml −1 leupeptin and 1 mM phenylmethylsulfonyl fluoride. The lysates were incubated with the glutathione S-transferase-rhotekin-Rho-binding domain previously bound to glutathione-Sepharose beads (Amersham Biosciences) and washed three times with lysis buffer. Associated GTP-bound forms of Rho were released with SDS–polyacrylamide gel electrophoresis loading buffer and analysed by western blot analysis using a monoclonal antibody against RhoA, as described above. Permeability assay Permeability was assessed by the passage of fluorescein isothiocyanate (FITC)-conjugated dextran (relative molecular mass 40,000; 1 mg ml −1 ; Molecular Probes) [10] . Immortal endothelial cells, 2 × 10 5 , were plated onto 6.5-mm Transwell Collagen-coated 3-μm pore polytetrafluoroethylene (PTFE) membrane inserts. Under these conditions, endothelial cells do not proliferate but form mature monolayers in around 3 days. When required, pools of 1 × 10 6 cells were first transfected and then distributed equally in inserts, and cell lysates were prepared in parallel for western blot analysis. Each sample was read on the Victor3 V, 14220 multilabel counter (Perkin-Elmer, Wellesley, MA) or the Synergy Neo HTS multi-mode microplate reader (BioTek, Winooski, VT). All data were expressed as ratio of FITC measurement of the tested drugs versus the control, and data from at least three independent experiments were quantified. Calcium measurement Calcium measurements were performed with the use of confocal microscopy [55] . Endothelial cells were grown onto collagen pre-coated glass-bottom microwell dishes (MatTek Corporation), were washed three times with a balanced Tyrode’s salt solution containing 5 mM Hepes, 136 mM NaCl, 2.7 mM KCl, 1 mM MgCl 2 , 1.9 mM CaCl 2 , 5.6 mM glucose, buffered to pH 7.4 with Tris base and supplemented with 0.1% BSA. The Fluo-3/AM probe was diluted in Tyrode-BSA to a final concentration of 6.5 μM, according to the manufacturer’s instructions. After a 45-min incubation period, the cells were washed twice with Tyrode-BSA buffer and twice in Tyrode buffer. Cells were monitored for 10 min after stimulation. In vivo permeability assay Agonist-induced vascular permeability changes were determined using Evans Blue dye (Miles assay) [56] . Five mice were anaesthetized by i.p. injections of ketamine (10 mg kg −1 ) and xylazine (100 mg kg −1 ) and were injected by intravenous (i.v.) injections sterile Evans Blue dye (100 μl, 1% in normal saline). After 1 min, different doses of histamine, PAF or VEGF in 20 μl PBS were injected into the shaved back skin. PBS was injected as control. Under these conditions, most agents causing vascular permeability promote the extravasation of Evans Blue within 3–5 min, reaching a maximum at ∼ 10–15 min [13] . Mice were euthanized after 10 min and ∼ 1 cm 2 of skin containing the site of injections was removed. The skin punches were incubated in 500 μl formamide at 55 °C for 48 h and the Evans Blue content was determined by absorption at 595 nm. Data were expressed as the ratio of the value of Evans Blue extravasation promoted by the tested substance versus the control injection (PBS) in the same mouse. All assays involving genetically defined mice were conducted using littermate controls. Passive cutaneous anaphylaxis Local anaphylactic response [20] was measured as follows: 30 ng of anti-DNP-IgE in 20 μl of sterile 0.9% NaCl were injected into the dorsal skin of the right ear. Six mice were used in each experiment. The left ear of mice received an equal volume of saline and served as control. After 24 h, the passively immunized mice were challenged by an i.v. injection of 0.5 mg of DNP-HSA together with 0.08 μg g −1 Evans Blue in normal saline. Mice were euthanized 30 min after the challenge and ear biopsies were collected. Evans Blue dye was extracted in 400 μl of formamide at 55 °C for 24 h and quantified by measuring light absorption at 595 nm. Active systemic anaphylaxis Active systemic anaphylaxis model was achieved as previously described [20] : five mice were immunized with i.p. injection of 1 mg BSA and 300 ng pertussis toxin as adjuvant in normal saline. After 14 days, mice were challenged with i.v. injection of 2 mg BSA. Survival of the mice was monitored for 120 min after the challenge. PAF-induced anaphylaxis The protocol for PAF-induced anaphylactic shock is the following [20] : seven mice were injected i.v. with 0.01 μg g −1 PAF and survival was monitored over 120 min. Immunofluorescence Monolayer-cultured human umbilical vein endothelial cells were plated on collagen-coated glass-base dishes and cultured for about 24 h. They were starved 3 h before the experiment with medium containing 0.5% BSA and then stimulated with histamine or VEGF. Immunofluorescence was performed as follows [57] : after stimulation, the cells were fixed with PBS containing 2% formaldehyde for 30 min at 4 °C, permeabilized with 0.05% Triton X-100 for 25 min at 4 °C and blocked with PBS containing 4% BSA for 1 h at room temperature. The cells were immunostained with anti-VE-cadherin, anti-vinculin and anti-pMLC primary antibodies at 4 °C overnight. Protein reacting with antibody was visualized with species-matched Alexa Fluor 488- or Alexa Fluor 633-labelled secondary antibodies. To visualize F-actin, the cells were stained with rhodamine-phalloidin for 1 h at room temperature. Fluorescence images of Alexa Fluor 488, Alexa Fluor 633 and rhodamine were recorded with an inverted fluorescence microscope (IX-81; Olympus) with Plan-Apochromat × 60/1.40 numerical aperture (NA) and UPlan FL N × 60/1.25 oil immersion objective lenses (Olympus) and equipped with a pE-1 LED excitation system (CoolLED) with a cooled charge-coupled device camera (CoolSNAP HQ; Roper Scienific) or with a confocal microscope (FluoView FV1000; Olympus) with UPlan-SApochromat × 60 1.35 NA oil immersion objective lens (Olympus). The microscope and image acquisition were controlled by MetaMorph software (Universal Imaging) and FluoView ASW software (Olympus). Trio-GFP plasma membrane translocation assays HEK 293 cells were grown onto pre-coated (poly- L -lysine) glass-bottom microwell dishes (MatTek Corporation). Cells were transfected with H1R1 and Trio-GFP. The next day, cells were serum starved for 4 h and incubated with CellMask Orange plasma membrane stain (Invitrogen) according to the manufacturer’s instructions. Cells were placed in the microscope in serum-free media and stimulated with histamine. To quantify the levels of Trio-GFP in the plasma membrane, the peak fluorescence value of a line histogram covering the plasma membrane region was recorded every 30 s and used to plot the fluorescent levels of membrane Trio over time. At least five different regions were quantified in a cell and averaged. Live cell imaging and quantifications were performed using an inverted Zeiss LSM 700 confocal microscope equipped with a temperature and CO 2 incubator, coupled to Zen software 2010 (Carl Zeiss). Intravital imaging of vascular leakage in mouse ear skin One day before the experiment, hair was removed from the imaging area by gently applying adhesive masking tape several times. The day of the experiment, the animals were anesthetized by i.p. injection of ketamine-xylazine in normal saline (ketamine 100 mg kg −1 and xylazine 10 mg kg −1 ). The mouse ear was stabilized on a customized ear-holder platform by adhering the ventral side to the adhesive masking tape using a moisten cotton tip. The masking tape was then stabilized onto the platform. Mouse was placed on heating pad with rectal temperature probe (TC-1000 Temperature controller, CEW-Inc.) to maintain body temperature of 37 °C throughout the imaging procedure. The blood vessels were labelled by intravenously injecting 500 kD FITC dextran (Molecular probe). Intravital microscopy was acquired using an inverted confocal microscope (model IX-81) Fluoview 1000 scanning head (Olympus America Inc., Center Valley, PA, USA) and the InverterScope objective Inverter for upright configuration (LSM technologies, Wellsville, PA). GFP and FITC dextran were excited with a 488-nm laser, whereas m-Tomato, TRITC were excited with a 561-nm laser. For time-lapse imaging of vascular leakage, mice were injected i.v. with 500 kDa FITC dextran and the ear skin was punched with a half-inch 29-gauge needle that had been embedded in 10 −4 M histamine solution. The acquisition speed was set to 1.64 frames per second. All images and movies were acquired using a UPLSAPO × 10, NA 0.4 objective and a XLPlanN × 25, NA 1.05 water immersion objectives with coupling gel (carbomer-940-based gel (Snowdrift Farm, Tucson, AZ)). The time series images were assembled using ImageJ (W. Rasband, National Institutes of Health) Brightness, contrast and gamma correction were applied. The montage images of time series were created using stack to montage function. Five different regions per picture were used for quantifications. Quantitative analysis of vascular leakage The vascular leakage after histamine administration was estimated from the change of average fluorescent intensity within the region of interest from ImageJ using Time series analyzer plugin V2.0. The measurement data were then transferred for statistical analysis. Statistical analysis All experiments were repeated at least three times with similar results. Statistical analysis was performed by an unpaired two-tailed Student’s t -test. Mantel–Cox test was used to quantify the difference in survival between control and treated groups. Data analysis was performed using GraphPad Prism version 4.00 for Windows (GraphPad Software, San Diego, CA). The asterisks in the figures denote statistical significance (not significant, P >0.05; * P <0.05; ** P <0.01; *** P <0.001). How to cite this article: Mikelis, C.M. et al . RhoA and ROCK mediate histamine-induced vascular leakage and anaphylactic shock. Nat. Commun. 6:6725 doi: 10.1038/ncomms7725 (2015).